klf2acouples mechanotransduction and zebrafish valve morphogenesis through fibronectin synthesis The heartbeat and blood flow signal to endocardial cell progenitors through mechanosensitive proteins that modulate the genetic program controlling heart valve morphogenesis. To date, the mechanism by which mechanical forces coordinate tissue morphogenesis is poorly understood. Here we use high-resolution imaging to uncover the coordinated cell behaviours leading to heart valve formation. We find that heart valves originate from progenitors located in the ventricle and atrium that generate the valve leaflets through a coordinated set of endocardial tissue movements. Gene profiling analyses and live imaging reveal that this reorganization is dependent on extracellular matrix proteins, in particular on the expression of fibronectin1b . We show that blood flow and klf2a , a major endocardial flow-responsive gene, control these cell behaviours and fibronectin1b synthesis. Our results uncover a unique multicellular layering process leading to leaflet formation and demonstrate that endocardial mechanotransduction and valve morphogenesis are coupled via cellular rearrangements mediated by fibronectin synthesis. Tissue morphogenesis and organ formation depend upon the cooperative behaviour of groups of cells as well as the integration of chemical inputs generated in growing tissues. In addition, cells experience environmental mechanical stresses, such as pressure, strain and shear stress, due to tissue deformation and biological flows [1] , [2] , which subsequently participate in driving morphogenetic movements [1] , [3] , [4] , [5] . Due to the early initiation of heart contraction, the formation of the cardiovascular system is intricately linked to its function. Indeed, flow forces are necessary for cardiac ballooning, trabeculation and epicardium formation with flow forces being necessary for cardiac ballooning [6] , trabeculation [7] , [8] and epicardium formation [9] . In both the lymphatic and cardiac systems, valves serve to maintain unidirectional fluid flow and, pertinently, depend on their respective flows to form [10] , [11] . Congenital heart valve malformations constitute an important medical issue challenging our society. In recent years, it has become clear that most valve disease has its origin during embryogenesis, either as signs of abnormal developmental processes or the aberrant re-expression of fetal gene programs normally quiescent in adulthood [12] , [13] . These include mutations in genes encoding signalling factors (Notch1 and TGFβ) [14] for the aortic valves, and actin-binding proteins (Filamin A) [15] for the mitral valves. Diseased valves often also display defects in extracellular matrix (ECM) deposition [16] , which plays an essential function in valve architecture [17] , [18] . Interestingly, studies of lymphatic valve formation have shown that the ECM proteins fibronectin and laminin are deposited during the initial stages of valve development [11] , [19] , implicating ECM deposition in the earliest stages of the valve-forming process. The complex three-dimensional (3D) shape and constant motion of the heart, however, make imaging the morphogenetic events during cardiac valve development particularly challenging, although live imaging approaches are being continuously pioneered to observe endothelial cell behaviours in their mechanically active context [20] , [21] , [22] , [23] . In the heart, the atrioventricular (AV) valve emanates from the endocardial wall and is composed of endocardial cells (EdCs) and ECM components [12] . While blood flow has a broad influence on the shape and growth of EdCs [6] , the oscillatory flow profile specific to the early AV canal (AVC) directs AV valve (AVV) formation by specifically increasing Krüppel-like factor 2a ( klf2a ) expression in the AVC [24] , [25] . As a transcription factor, klf2a expression likely allows EdCs to couple mechanotransduction to valve morphogenesis by activating a range of downstream target genes. The identity of such Klf2a target genes in valve-forming EdCs and the subsequent cellular behaviours induced, however, are unknown. In this study, we investigated the cellular events taking place during valve formation and addressed their regulation by the flow-responsive transcription factor Klf2a. We show that valve formation proceeds via an initial stage of cell clustering followed by the appearance of cellular extensions towards the cardiac jelly. Subsequent global tissue remodelling events result in the appearance of ventricular and AVC-derived EdCs in the cardiac jelly overlying atrial-derived EdCs exposed to the lumen. Using transcriptomic analyses to highlight the transcriptional changes accompanying these temporally coordinated cell-movement events, we identified fibronectin1b as a key Klf2a- and flow-dependent factor necessary for the correct coordination of valvulogenesis. These data describe cell behaviour that is coordinated by the mechanical environment and mechanotransduction via Klf2a and ECM deposition. Endocardial cell contributions to the atrioventricular valve AVV morphogenesis begins ∼ 48 hours post fertilization (hpf). By 5 days post fertilization (dpf) a set of functional valve leaflets, extend into the AVC, occluding the passage of reversing blood flow [26] , [27] , [28] . To uncover the origins of the EdCs contributing to the AVV, we performed photoconversion experiments using the Tg(fli1a:Gal4FF ubs , UAS:kaede) transgenic line, in which the photoconvertible protein kaede is expressed in the endothelial cells, including the endocardium. The exposure of kaede to 405 nm light results in an irreversible fluorescence conversion from fluorescent green to fluorescent red, enabling the development of cells labelled with the red form to be followed with respect to their green neighbours during AVV formation. As EdCs of the AVC can be identified by their positivity for Alcama [26] , we used our knowledge of this staining pattern ( Fig. 1a ) to specifically photoconvert green kaede to its red form in the atrium and ventricle at 48 hpf. We then focused on the subsequent development of the superior AVC as it undergoes valve morphogenesis earlier than the inferior AVC [26] . Heart contraction was temporarily blocked using 2,3-butanedione-2-monoxime (BDM) to enable the photoconversion to be performed. Following photoconversion, heart contraction was resumed and embryos were allowed to develop under standard conditions until imaging at 80 hpf, enabling us to assess the contribution of EdCs from each region to the forming superior AVV leaflet ( Fig. 1b ). Atrial cells photoconverted at 48 hpf were seen lining the AVC lumen at 80 hpf ( Fig. 1c ), and were never present inside the cardiac jelly following the formation of multiple cell layers ( n =12/12). In contrast, photoconversion of cells in the ventricular region of the superior AVC at 48 hpf resulted in photoconverted cells in the cardiac jelly at 80 hpf ( n =7/7 Fig. 1d ). When ventricular photoconversion was performed away from the ventricular inner curvature, no photoconverted cells were observed inside the cardiac jelly ( n =3/3; Fig. 1e ). Thus, in addition to the cells of the AVC, EdCs from the atrium and ventricular inner curvature make significant and distinct contributions to the forming valve leaflets at 80 hpf ( Fig. 1f ). Furthermore, these distinct contributions are maintained at 120 and 168 hpf, suggesting mixing of cells from atrial and ventricular origins does not occur in the AVV at later stages ( Supplementary Fig. 1 ). These findings implicate the ventricle and atrium as important sources of valve progenitors and suggest that stereotyped and coordinated cellular behaviours guide valve morphogenesis. 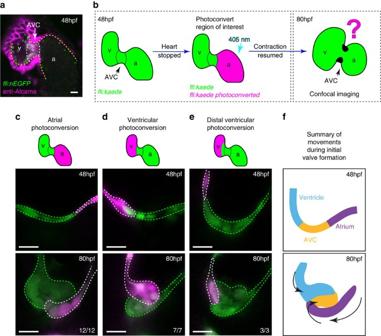Figure 1: The cellular contribution of heart chambers to emerging valve leaflets. (a) anti-Alcama immunofluorescence analysis shows Alcama-positive EdCs in the AVC offli:nEGFPhearts (white dotted line), used to define the cardiac chambers at 48 hpf. Yellow dashed line delineates the endocardium from the myocardium, which also stains positively for Alcama. v=ventricle, a=atrium, AVC=atrioventricular canal. (b) The experimental set-up for the photoconversion studies. Heart contraction was stopped infli:kaedeembryos at 48 hpf, the region of interest exposed to 405 nm light to convert kaede from a green to red (shown here to be the atrium, in magenta) fluorescent form and heart contraction was then resumed until 80 hpf. Stopped hearts were imaged at 80 hpf by confocal microscopy. (c) EdCs present in the atrium and Alcama-negative at 48 hpf lined the lumen of the AVC at 80 hpf (n=12/12, 3 experiments), while those in the ventricle contribute cells to the cardiac jelly (d;n=7/7, 3 experiments). Ventricular cells outside the ventricular inner curvature (distal ventricle) do not enter the cardiac jelly at 80 hpf (e;n=3/3, 2 experiments). In all cases only the superior valve leaflet is shown. (f) Schematic representation of the cellular contributions of each chamber to the emerging valve leaflet at 80 hpf. Atrial cells (purple) line the lumen of the AVC, while EdCs originating in the ventricular inner curvature (blue) and AVC (yellow) contribute cells to the cardiac jelly. Black arrows highlight the coordinated movements of the groups of cells. Scale bars, 10 μm. Figure 1: The cellular contribution of heart chambers to emerging valve leaflets. ( a ) anti-Alcama immunofluorescence analysis shows Alcama-positive EdCs in the AVC of fli:nEGFP hearts (white dotted line), used to define the cardiac chambers at 48 hpf. Yellow dashed line delineates the endocardium from the myocardium, which also stains positively for Alcama. v=ventricle, a=atrium, AVC=atrioventricular canal. ( b ) The experimental set-up for the photoconversion studies. Heart contraction was stopped in fli:kaede embryos at 48 hpf, the region of interest exposed to 405 nm light to convert kaede from a green to red (shown here to be the atrium, in magenta) fluorescent form and heart contraction was then resumed until 80 hpf. Stopped hearts were imaged at 80 hpf by confocal microscopy. ( c ) EdCs present in the atrium and Alcama-negative at 48 hpf lined the lumen of the AVC at 80 hpf ( n =12/12, 3 experiments), while those in the ventricle contribute cells to the cardiac jelly ( d ; n =7/7, 3 experiments). Ventricular cells outside the ventricular inner curvature (distal ventricle) do not enter the cardiac jelly at 80 hpf ( e ; n =3/3, 2 experiments). In all cases only the superior valve leaflet is shown. ( f ) Schematic representation of the cellular contributions of each chamber to the emerging valve leaflet at 80 hpf. Atrial cells (purple) line the lumen of the AVC, while EdCs originating in the ventricular inner curvature (blue) and AVC (yellow) contribute cells to the cardiac jelly. Black arrows highlight the coordinated movements of the groups of cells. Scale bars, 10 μm. Full size image Cell density and protrusive activity in early valvulogenesis To elucidate how cells of the atrium and ventricle reorganize to contribute to the developing valve leaflets, we characterized the organization of EdCs in the AVC in the moments preceding the appearance of multiple cell layers, beginning at 36 hpf. Using Tg(fli:nlsmCherry) embryos, in which the EdC nuclei are labelled, we observed nuclei to be relatively evenly spaced around the AVC at 36 hpf, before undergoing regional increases in cell density at 48 hpf ( Fig. 2a–d and Supplementary Movie 1 ). Quantification of total cell numbers in the AVC showed a doubling of EdCs in the AVC between 36 and 48 hpf, ( Fig. 2b ). Photoconversion experiments suggest that cells move towards the AVC from the atrium between 36 and 48 hpf, while ventricular cells maintain their position at the ventricular inner curvature/exit of the AVC ( Supplementary Fig. 2 ). In the absence of multi-layering, at this stage, this results in an increased density of cells within the AVC, particularly on the ventricular side. Incubation of embryos in BrdU between these stages demonstrated that ∼ 60% of the atrial cells and ∼ 40% of the cells from both the ventricle and the AVC proliferate during this time ( Supplementary Fig. 2E,F ), suggesting cell proliferation throughout the heart could be an important contributing factor to the increased cell density observed in the AVC at 48 hpf. Visualization of the superior leaflet alone enabled the changes in cell density between 36 and 48 hpf to be seen more clearly ( Fig. 2c,d ). A region of increased cell density was particularly apparent on the ventricular side of the superior AVC at 48 hpf, containing 11±3 cells ( n =5). The numbers of cells in this clustered region stayed the same at 56 hpf (11±2 cells; n =5; Fig. 2d and Supplementary Movie 2 ). Quantification of distances between neighbouring nuclei at these stages confirmed cells in the clustered region were indeed more closely packed together than those around the rest of the AVC ( Fig. 2e and see Supplementary Movie 3 ) suggesting regional increases in cell density accompany the increases in cell numbers observed. 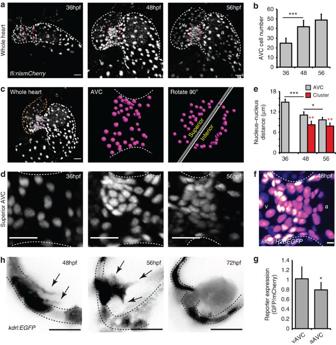Figure 2: EdCs move into the cardiac jelly from a region of increased cell density. (a)fli:nlsmCherryhearts imaged at early stages of heart development show the organization of EdCs between 36 and 56 hpf. White dotted lines outline the endocardium. Magenta dotted lines mark the AVC. (b) Total AVC cell number quantification at 36, 48 and 56 hpf. (c) Demonstration of how the superior AVC is defined and presented ind: The nuclei of AVC EdCs are defined (magenta spots) from images of the whole heart (orange/v= ventricle; white/a=atrium), rotated 90 °C using Imaris software and then divided into two parts, the superior AVC (to be the upper leaflet) and the inferior AVC (to be the lower leaflet). Orthogonal views of the superior AVC are then shown to display nuclei organization ind. (d) Regional increases in cell density can be seen on the ventricular side of the AVC from 48 hpf (n=5 at each developmental stage). (e) Quantification of nucleus-nucleus distances within the AVC shows enhanced proximity of nuclei within the cluster region. No red bar at 36 hpf signifies the absence of a cluster at this stage. (f)klf2aexpression pattern in the whole AVC at 48 hpf in theklf2a:H2BEGFPtransgenic line shows enrichment of GFP signal on the ventricular side. The GFP signal is shown as FireLUT to aid visualization (white=highest intensity, black=no signal). (g) Relative reporter expression level in the ventricular (vAVC) and atrial (aAVC) regions of the AVC (n=10). (h) Imaging ofkdrl:EGFPhearts demonstrates the presence of protrusions (black arrows) extending from the region of clustered cells towards the cardiac jelly at 48 hpf. Cells emanating into the cardiac jelly can be seen from 56 hpf. Protrusions are also still visible (black arrows). Groups of cells are present in the cardiac jelly by 72 hpf. Inverted images of thekdrl:EGFPsignal are shown to aid visualization of the protrusive structures. Black dotted lines mark the EdCs layer. Error bars in all graphs represent the s.d. Student’st-test ***P<0.005, **P<0.01, *P<0.05. Scale bars, 10 μm; except inf: 2 μm. Figure 2: EdCs move into the cardiac jelly from a region of increased cell density. ( a ) fli:nlsmCherry hearts imaged at early stages of heart development show the organization of EdCs between 36 and 56 hpf. White dotted lines outline the endocardium. Magenta dotted lines mark the AVC. ( b ) Total AVC cell number quantification at 36, 48 and 56 hpf. ( c ) Demonstration of how the superior AVC is defined and presented in d : The nuclei of AVC EdCs are defined (magenta spots) from images of the whole heart (orange/v= ventricle; white/a=atrium), rotated 90 °C using Imaris software and then divided into two parts, the superior AVC (to be the upper leaflet) and the inferior AVC (to be the lower leaflet). Orthogonal views of the superior AVC are then shown to display nuclei organization in d . ( d ) Regional increases in cell density can be seen on the ventricular side of the AVC from 48 hpf ( n =5 at each developmental stage). ( e ) Quantification of nucleus-nucleus distances within the AVC shows enhanced proximity of nuclei within the cluster region. No red bar at 36 hpf signifies the absence of a cluster at this stage. ( f ) klf2a expression pattern in the whole AVC at 48 hpf in the klf2a:H2BEGFP transgenic line shows enrichment of GFP signal on the ventricular side. The GFP signal is shown as FireLUT to aid visualization (white=highest intensity, black=no signal). ( g ) Relative reporter expression level in the ventricular (vAVC) and atrial (aAVC) regions of the AVC ( n =10). ( h ) Imaging of kdrl:EGFP hearts demonstrates the presence of protrusions (black arrows) extending from the region of clustered cells towards the cardiac jelly at 48 hpf. Cells emanating into the cardiac jelly can be seen from 56 hpf. Protrusions are also still visible (black arrows). Groups of cells are present in the cardiac jelly by 72 hpf. Inverted images of the kdrl:EGFP signal are shown to aid visualization of the protrusive structures. Black dotted lines mark the EdCs layer. Error bars in all graphs represent the s.d. Student’s t -test *** P <0.005, ** P <0.01, * P <0.05. Scale bars, 10 μm; except in f : 2 μm. Full size image We recently demonstrated the sensitivity of EdCs in detecting flow forces and inducing the expression of the flow-responsive transcription factor klf2a (ref. 24 ). In light of this, we investigated the distribution of klf2a expressing cells, more specifically, within the AVC. Using a klf2a reporter line ( Tg(klf2a:H2BEGFP) [24] , we observed higher levels of GFP expression in those nuclei closest to the ventricle, compared with those on the atrial side of the AVC ( Fig. 2f,g ), corresponding to the region of cell clustering. Interestingly, protrusions were observed emanating from EdCs in this region towards the cardiac jelly at 48 hpf ( Fig. 2h and Supplementary Movie 4 ). By 56 hpf, cells could be observed extending further into the cardiac jelly and by 72 hpf multiple layers of cells were present. To confirm the relevance of these observations in the beating heart, we performed fast confocal imaging of Tg(kdrl:EGFP) embryos and observed the same arrangement of cells at 72 hpf ( n =3; Supplementary Movie 5 ). Indeed when the heart is contracting, the connection of the EdCs within the cardiac jelly to the region of the heart wall from where they originate is clear ( Supplementary Movie 5 ). These observations enable us to describe, for the first time, a cluster of EdCs close to the ventricular inner curvature at 48 hpf, from which cellular protrusions and movement of cells into the cardiac jelly originates. Cardiac jelly cells present distinct characteristics Analysis of the Tg(kdrl:EGFP) line at 80 hpf showed cells in the cardiac jelly to have a distinct mesenchymal-like morphology in comparison with those exposed to the lumen ( Fig. 3a ). Closer inspection of AVC morphology highlighted a deformation in the endocardial wall towards the cardiac jelly, which was wider towards the centre of the AVC ( Fig. 3a–d ). This morphology suggests a bending of the endocardial wall in response to the localized movement of EdCs into the cardiac jelly. In keeping with their mesenchymal-like morphology, junctional Cdh5 (VE-Cadherin) was lost between the neighbouring cells in the cardiac jelly at 72 hpf ( Fig. 3e ). Interestingly, BrdU-incorporation assays revealed the presence of BrdU-positive cells in the cardiac jelly, but not in the AVC wall between 56–72 hpf and 72–80 hpf ( Fig. 3f and g ). This suggests EdCs proliferate in the cardiac jelly, but do not enter it as a result of asymmetric cell division. Finally, analysis of klf2a reporter activity at 80 hpf, after multi-layering, showed EdCs exposed to the lumen expressed higher levels of klf2a activity than those in the cardiac jelly ( Fig. 3h,i ). This suggests klf2a is not continuously expressed in the EdCs that undergo multi-layering, as they originate in the region of the AVC where klf2a expression is high and then enter the cardiac jelly where klf2a expression is low. Furthermore, cells originally expressing low levels of klf2a in the atrium [24] appear to initiate klf2a expression upon entering the AVC. These observations define two subsets of cells within the AVC following multi-layering; one klf2a low , Cdh5 low , proliferative population within the cardiac jelly overlying a second klf2a high , Cdh5 high population exposed to the blood flow. On the basis of these observations we propose a model to describe the early cellular events involved in AVV formation ( Fig. 3j ). EdCs cluster in a region of the AVC close to the ventricular inner curvature at 48 hpf, corresponding to the region of increased klf2a expression. EdCs in this clustered region extend protrusions and emanate into the cardiac jelly, initiating the coordinated morphogenetic movements that result in multiple layers of EdCs within the cardiac jelly by 80 hpf. Once inside the cardiac jelly, EdCs display a mesenchymal-like phenotype with reduced levels of Cdh5 and klf2a , and increased proliferation. 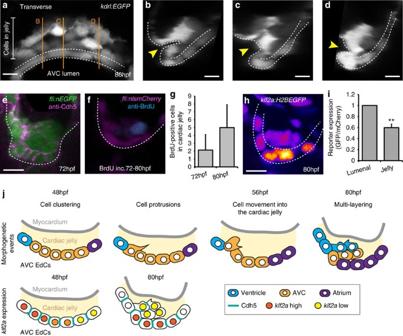Figure 3: EdCs display distinct characteristics inside the cardiac jelly. (a) Transverse section of akdrl:EGFPAVC at 80 hpf shows distinctive cell shapes within the AVC. Cells in the cardiac jelly have a mesenchymal morphology compared with those lining the lumen (enclosed in white dotted lines). Orange lines mark the positions of images i–iii. (b–d) white dotted line outlines the luminal EdCs and the yellow arrowheads highlight the deformation of the ventricular wall towards the cardiac jelly. The protrusive morphology of the cells within the cardiac jelly can also be observed. (e) Immunofluorescence analysis shows downregulation of Cdh5 between EdCs in the cardiac jelly (n=9). (f) anti-BrdU immunofluorescence following BrdU incubation between 72–80 hpf shows a BrdU-positive cell in the cardiac jelly. Shown is a singlezslice. (g) Quantification of total numbers of BrdU-positive cells in the cardiac jelly at 72 hpf (BrdU incubation=56–72 hpf;n=7) and 80 hpf (BrdU incubation=72–80 hpf;n=5) (h) Imaging of theklf2a:H2BEGFPreporter line shows theklf2aexpression pattern in the AVC at 80 hpf (GFP signal shown as FireLUT). (i) Normalized relative reporter expression levels in the EdCs exposed to the AVC lumen (lumenal) and those inside the cardiac jelly (jelly) (all cells in the superior AVC analysed from three embryos). Error bar represents the standard deviation. **P<0.01. (j) Model of the early stages of AVV formation. In the first series, cells are colour-coded to describe the morphogenetic events occurring during valve formation. Cells originating in the atrium (purple), AVC (yellow) and ventricle (blue) at 48 hpf and their relative positions at 80 hpf are shown. In the second series, Cdh5 andklf2alevels within the AVC are represented for the time points assessed. The myocardium is shown in grey and the cardiac jelly in pale yellow. Descriptions of the key stages at the relevant developmental time points are noted. Student’st-test ***P<0.005, **P<0.01, *P<0.05. Scale bars, 10 μm. Figure 3: EdCs display distinct characteristics inside the cardiac jelly. ( a ) Transverse section of a kdrl:EGFP AVC at 80 hpf shows distinctive cell shapes within the AVC. Cells in the cardiac jelly have a mesenchymal morphology compared with those lining the lumen (enclosed in white dotted lines). Orange lines mark the positions of images i–iii. ( b – d ) white dotted line outlines the luminal EdCs and the yellow arrowheads highlight the deformation of the ventricular wall towards the cardiac jelly. The protrusive morphology of the cells within the cardiac jelly can also be observed. ( e ) Immunofluorescence analysis shows downregulation of Cdh5 between EdCs in the cardiac jelly ( n =9). ( f ) anti-BrdU immunofluorescence following BrdU incubation between 72–80 hpf shows a BrdU-positive cell in the cardiac jelly. Shown is a single z slice. ( g ) Quantification of total numbers of BrdU-positive cells in the cardiac jelly at 72 hpf (BrdU incubation=56–72 hpf; n =7) and 80 hpf (BrdU incubation=72–80 hpf; n =5) ( h ) Imaging of the klf2a:H2BEGFP reporter line shows the klf2a expression pattern in the AVC at 80 hpf (GFP signal shown as FireLUT). ( i ) Normalized relative reporter expression levels in the EdCs exposed to the AVC lumen (lumenal) and those inside the cardiac jelly (jelly) (all cells in the superior AVC analysed from three embryos). Error bar represents the standard deviation. ** P <0.01. ( j ) Model of the early stages of AVV formation. In the first series, cells are colour-coded to describe the morphogenetic events occurring during valve formation. Cells originating in the atrium (purple), AVC (yellow) and ventricle (blue) at 48 hpf and their relative positions at 80 hpf are shown. In the second series, Cdh5 and klf2a levels within the AVC are represented for the time points assessed. The myocardium is shown in grey and the cardiac jelly in pale yellow. Descriptions of the key stages at the relevant developmental time points are noted. Student’s t -test *** P <0.005, ** P <0.01, * P <0.05. Scale bars, 10 μm. Full size image Transcriptional changes in early valvulogenesis To elucidate how these early events are regulated, we sought to determine the gene expression profile activated at these early stages of valve formation. To do so, we extracted RNA from hearts dissected from 48 and 56 hpf myl7:EGFP embryos and performed transcriptome analysis using an Illumina sequencing platform ( Fig. 4a ). Between 31 and 65 million reads were generated for each RNA sample, of which, on an average, 67% could be mapped onto the Zv9 assembly of the zebrafish genome. We identified 1,628 genes that were significantly, differentially expressed in the heart between 48 and 56 hpf (FDR<0.05). Importantly, we saw a downregulation of has2 and an upregulation of klf2a , confirming the reliability of our approach ( Fig. 4b ). Real-time quantitative PCR (qPCR) analysis of heart RNA confirmed the respective up and downregulation of these genes with time ( Fig. 4c ). Considering only those genes with a logFC>1, we found 1,076 genes to be upregulated during these early stages of valve development. To assess the biological significance of these genes, we then performed Gene Ontology analysis using DAVID software [29] . By clustering genes based on cellular compartment annotations we saw a strong enrichment for ECM protein terms ( Fig. 4d ). Closer analysis of the 31 genes found in the ‘extracellular region’ term demonstrated that, among others, fibronectin1b was significantly upregulated in the heart between 48 and 56 hpf ( Fig. 4e ). Given the importance of fibronectin deposition in lymph valve formation [19] , we questioned whether it could also play a role in AVV formation. qPCR analysis of heart-derived RNA showed fibronectin1b is indeed expressed in the heart during this period of its development and confirmed the increase of transcript levels between 48 and 56 hpf ( Fig. 4f ). We next addressed the temporal and spatial expression of fibronectin within the heart at the protein level through immunofluorescence analysis. Interestingly, fibronectin protein is expressed specifically in the AVC at 48 hpf ( Fig. 4g ) with further enrichment by 56 hpf, in keeping with the mRNA sequencing data ( Fig. 4h ). More specifically, fibronectin is seen on the basal side of cells at both time points and is particularly enriched in the region of cell clustering ( Fig. 4g,h ). Fibronectin can also be observed on and between the multiple layers of cells that are present by 72 hpf ( Fig. 4i ), as has previously been shown in 105 hpf hearts [26] . This spatial and temporal expression pattern in the heart suggests a potentially relevant role of fibronectin1b /fibronectin in cardiac valve development. 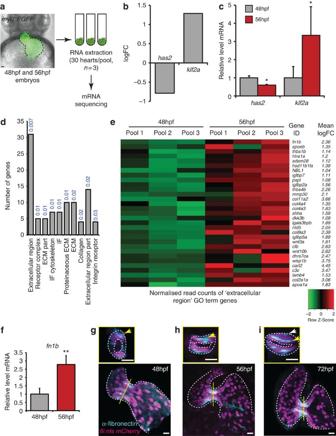Figure 4: Transcriptome analysis identifies increased ECM protein gene expression during initial stages of valve formation. (a) Experimental set-up for mRNA sequencing. RNA was extracted from hearts ofmyl7:EGFPembryos dissected at 48 and 56 hpf, in pools of 30 (n=3). (b) Downregulation ofhas2and upregulation ofklf2atranscripts, confirmed by qPCR (c), validated our approach. (d) Gene Ontology (GO) analysis based on cellular compartment terms of upregulated genes highlighted a significant enrichment of ECM-related terms.Pvalues describing the significance of each term enrichment are shown in blue. (e) Specific analysis of the most significantly enriched group (the ‘extracellular region’ term), highlighting, among others, elevated fibronectin1b expression between 48 and 56 hpf. (f) qPCR analysis of heart RNA confirms an increase in fn1b transcript levels between 48 and 56 hpf. (g–i) Immunofluorescence analysis shows fibronectin synthesis is localized to the AVC during early stages of valve formation (n=8 (48 hpf),n=11 (56 hpf) andn=7 (72 hpf)). Yellow lines mark the position of the transverse sections shown in small panels. Yellow arrows highlight enriched fibronectin-positive staining in the superior AVC. White arrow in small panel (i) points to fibronectin deposition on multiple cell layers. Student’st-test ***P<0.005, **P<0.01, *P<0.05. Scale bars, 10 μm. Figure 4: Transcriptome analysis identifies increased ECM protein gene expression during initial stages of valve formation. ( a ) Experimental set-up for mRNA sequencing. RNA was extracted from hearts of myl7:EGFP embryos dissected at 48 and 56 hpf, in pools of 30 ( n =3). ( b ) Downregulation of has2 and upregulation of klf2a transcripts, confirmed by qPCR ( c ), validated our approach. ( d ) Gene Ontology (GO) analysis based on cellular compartment terms of upregulated genes highlighted a significant enrichment of ECM-related terms. P values describing the significance of each term enrichment are shown in blue. ( e ) Specific analysis of the most significantly enriched group (the ‘extracellular region’ term), highlighting, among others, elevated fibronectin1b expression between 48 and 56 hpf. ( f ) qPCR analysis of heart RNA confirms an increase in fn1b transcript levels between 48 and 56 hpf. ( g – i ) Immunofluorescence analysis shows fibronectin synthesis is localized to the AVC during early stages of valve formation ( n =8 (48 hpf), n =11 (56 hpf) and n =7 (72 hpf)). Yellow lines mark the position of the transverse sections shown in small panels. Yellow arrows highlight enriched fibronectin-positive staining in the superior AVC. White arrow in small panel ( i ) points to fibronectin deposition on multiple cell layers. Student’s t -test *** P <0.005, ** P <0.01, * P <0.05. Scale bars, 10 μm. Full size image Blood flow and klf2a alter fibronectin synthesis in the AVC As blood flow is an important regulator of EdC behaviour and cardiac valve formation, we next wanted to assess whether changes in flow properties impacted fibronectin synthesis in the AVC. To do so, we first analysed the fibronectin staining pattern in silent heart ( sih −/− ) mutant embryos, which completely lack heart contraction and blood flow [30] , and saw that fibronectin was no longer detectable in the AVC at 48 hpf ( Fig. 5a ). As sih −/− mutants fail to form an AVV, we performed photoconversion experiments following injection of a morpholino specific for troponin T2a ( tnnt2a ), which is necessary for heart contraction and reliably mimics the sih −/− mutants [30] , to determine whether the cell-movement events described above were impacted in the absence of heart contraction. Indeed, in tnnt2a MO hearts at 80 hpf, the photoconverted cells were found on the inner curvature of the ventricle and had failed to enter the cardiac jelly, as observed in age-matched controls ( Supplementary Fig. 3A,B ). To address the role of flow forces more specifically, we then altered blood viscosity and shear stress by lowering haematocrit content by injecting gata1 and gata2 morpholinos, as previously described [25] . In gata1 morphants, where the fraction of reversing flow in the AVC at 48 hpf is increased and klf2a expression is high [24] , strong fibronectin staining was observed in the AVC ( Fig. 5b ), while it was much reduced or absent in gata2 morphants where the fraction of reversing flow in the AVC, and klf2a expression, is reduced ( Fig. 5b ). When atrial contraction was affected in myh6 morphants (atrial specific myosin heavy chain, previously amhc ), which also results in reduced klf2a expression [31] ( Supplementary Fig. 3E,F ), fibronectin deposition was also impaired ( n =6/7; Fig. 5b ). Quantification of the proportion of the AVC positive for fibronectin confirmed these observations ( Fig. 5c ). Furthermore, fibronectin synthesis was significantly reduced, compared with controls, when 0.1% tricaine was used to stop heart contraction between 48 and 52 hpf and between 48 and 56 hpf ( Fig. 5d ). Interestingly, when the 0.1% tricaine was removed and heart contraction resumed at 52 hpf, fibronectin staining in the AVC at 56 hpf was restored ( Fig. 5d,e ). Taken together these observations suggest that the synthesis of fibronectin in the AVC is flow-dependent. To ascertain how conditions of altered flow may impact cellular organization during valve formation, we repeated our photoconversion experiments in the flow morphants described above. We observed cells in the cardiac jelly of gata1 MO embryos, but this was greatly reduced in gata2 MO and absent in myh6 MO embryos, when compared with controls ( Supplementary Fig. 3C,D ). Furthermore, in gata1 MOs, cells in the cardiac jelly appeared to be more disorganized than in controls ( Supplementary Fig. 3C,D ) suggesting AVC-specific fibronectin synthesis may be necessary for the correct organization of multiple cell layers before leaflet emanation. 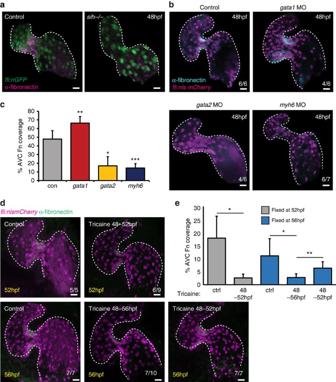Figure 5: AVC-specific fibronectin synthesis is dependent on blood flow forces. (a) Fibronectin staining (magenta) is lost in the absence of heart contraction (fli:nEGFP, sih−/−embryos) (n=6/6). (b)fli:nlsmCherryembryos injected withgata1,gata2ormyh6morpholinos to alter blood flow forces were fixed at 48 hpf and anti-fibronectin immunofluorescence analysis was performed. Alterations in flow forces impacted fibronectin synthesis (cyan) in the AVC ofgata1,gata2ormyh6morphants. (c) Quantification of extent of fibronectin (Fn)-positive staining confirms an increase ingata1morphants and a reduction in bothgata2andmyh6morphants. (d) fli:nlsmCherry(magenta) embryos were incubated with 0.1% tricaine between 48–52 and 48–56 hpf to stop heart contraction. When necessary, heart contraction was restored at 52 hpf by washing out tricaine and embryos were left to develop under normal conditions until 56 hpf. Yellow font shows embryonic age at fixation. Anti-fibronectin immunofluorescence (green) shows the flow-responsive nature of fibronectin in the AVC. (e) Quantification of extent of fibronectin-positive staining confirms the restoration of fibronectin synthesis following restoration of heart contraction. Control (ctrl) samples were not incubated in 0.1% tricaine. Student’st-test ***P<0.005, **P<0.01, *P<0.05. Scale bars, 10 μm. Figure 5: AVC-specific fibronectin synthesis is dependent on blood flow forces. ( a ) Fibronectin staining (magenta) is lost in the absence of heart contraction ( fli:nEGFP, sih −/− embryos) ( n =6/6). ( b ) fli:nlsmCherry embryos injected with gata1 , gata2 or myh6 morpholinos to alter blood flow forces were fixed at 48 hpf and anti-fibronectin immunofluorescence analysis was performed. Alterations in flow forces impacted fibronectin synthesis (cyan) in the AVC of gata1 , gata2 or myh6 morphants. ( c ) Quantification of extent of fibronectin (Fn)-positive staining confirms an increase in gata1 morphants and a reduction in both gata2 and myh6 morphants. ( d ) fli:nlsmCherry (magenta) embryos were incubated with 0.1% tricaine between 48–52 and 48–56 hpf to stop heart contraction. When necessary, heart contraction was restored at 52 hpf by washing out tricaine and embryos were left to develop under normal conditions until 56 hpf. Yellow font shows embryonic age at fixation. Anti-fibronectin immunofluorescence (green) shows the flow-responsive nature of fibronectin in the AVC. ( e ) Quantification of extent of fibronectin-positive staining confirms the restoration of fibronectin synthesis following restoration of heart contraction. Control (ctrl) samples were not incubated in 0.1% tricaine. Student’s t -test *** P <0.005, ** P <0.01, * P <0.05. Scale bars, 10 μm. Full size image AVC-specific fibronectin synthesis is necessary for valve formation Considering the apparent flow-dependent nature of fibronectin synthesis in the AVC and its increased levels on the ventricular side of the superior AVC, where klf2a is most highly expressed, we reasoned that fibronectin1b could be a downstream target of Klf2a. As klf2a is elevated in response to the specific flow regime found within the AVC [24] , such a target would enable klf2a to both respond to the mechanical environment of the AVC and impact the local environment of EdCs in a manner necessary for valve formation. Indeed, fibronectin staining was reduced in trpp2 −/− mutants ( Fig. 6a ), which present defects in valvulogenesis and klf2a induction despite a normal flow regime in the AVC [24] . To address the effect of loss of klf2a and validate previous observations performed using morpholino-based approaches, we generated a mutant of klf2a using a TALEN approach targeting a sequence in the first exon of the klf2a gene ( Supplementary Fig. 4A ). Observations of valve morphology at 96 hpf, when valve leaflets can be seen extending into the lumen of the AVC in controls, demonstrated a range of valvular defects in klf2a mutants ( Fig. 6b,c ; n =25 wild-type, n =46 klf2a −/− ) despite there being no change in overall cell numbers ( Supplementary Fig. 4B ) or flow properties ( Supplementary Fig. 4E ) at 48 hpf. Approximately 10% of klf2a −/− embryos were missing any kind of valve structure. Identical analyses performed in klf2a morpholino-injected embryos showed a similar, but more severe, phenotype in the knock down ( Fig. 6c ) and all subsequent studies were performed with the klf2a mutant. To investigate origins of the valve defects observed in the klf2a −/− mutants, we examined these embryos during the early stages of valve formation described above. Analysis of cell organization showed klf2a −/− embryos had fewer cells clustering together in the superior AVC at 48 hpf than controls ( Supplementary Fig. 4C ). Quantification of cells within the cardiac jelly suggested multi-layering was impaired in ∼ 40% of klf2a −/− hearts while the remaining klf2a −/− hearts presented elevated numbers of EdCs in the cardiac jelly at 72 hpf when compared with controls ( Fig. 6d and Supplementary Fig. 4D ). In those mutants where multi-layering occurred, however, the cells in the cardiac jelly appeared disorganized, with intracellular spaces between neighbouring EdCs, compared with the compact nature of the cells in this area in controls ( Fig. 6d,e and Supplementary Movie 6 ). These data suggest that, in the absence of klf2a function, the cellular processes underlying the initiation of valve formation are perturbed and support observations made with klf2a morpholinos that klf2a expression is necessary for efficient valvulogenesis [25] . 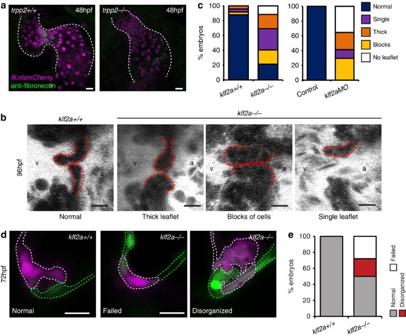Figure 6: Characterization ofklf2a−/−mutants. (a) anti-fibronectin staining (green) is reduced in the AVC oftrpp2−/−mutants (12/12trpp2+/+, 9/19trpp2−/−). (b,c) A range of valvular defects were observed inklf2a−/−mutant embryos at 96 hpf (n=25klf2a+/+,n=48klf2a−/−), similar to those observed inklf2aMO-injected embryos (e;n=20 control,n=17klf2aMO). (d) Photoconversion of AVC EdCs at 48 hpf shows the organization of cells within the cardiac jelly to be affected by loss ofklf2a(d,e;n=21klf2+/+,n=32klf2a−/−) at 72 hpf. Scale bars, 10 μm. Figure 6: Characterization of klf2a −/− mutants. ( a ) anti-fibronectin staining (green) is reduced in the AVC of trpp2 −/− mutants (12/12 trpp2 +/+ , 9/19 trpp2 −/− ). ( b , c ) A range of valvular defects were observed in klf2a −/− mutant embryos at 96 hpf ( n =25 klf2a +/+ , n =48 klf2a −/− ), similar to those observed in klf2a MO-injected embryos ( e ; n =20 control, n =17 klf2a MO). ( d ) Photoconversion of AVC EdCs at 48 hpf shows the organization of cells within the cardiac jelly to be affected by loss of klf2a ( d , e ; n =21 klf2 +/+ , n =32 klf2a −/− ) at 72 hpf. Scale bars, 10 μm. Full size image In situ hybridization and immunofluorescence analysis demonstrated that fibronectin is downregulated at both the mRNA and protein level in the majority of klf2a mutants ( Fig. 7a,b ). Furthermore, when we forced the overexpression of klf2a in all endothelial cells, we saw a spread of fibronectin synthesis outside the AVC, into the atrium and ventricle, in comparison with the AVC-specific localization observed in controls ( Fig. 7c ). This suggests that Klf2a, the expression of which is normally restricted to the AVC, is capable of driving the expression of fibronectin in the heart. Indeed, forced expression of klf2a was sufficient to rescue fibronectin synthesis in gata2 and myh6 morphant embryos ( Supplementary Fig. 5G ). To quantify the efficacy of valve progenitors in undergoing multi-layering in the absence of fibronectin, a vital process in the formation of the heart valve, we used a fn1b -specific morpholino to deplete fibronectin in the AVC ( Supplementary Fig. 5A ). Care was taken to select embryos presenting no morphological defects following fn1b MO injection ( Supplementary Fig. 5B ), ensuring that klf2a reporter activity, AVC cell number and the flow velocity profile at 48 hpf ( Supplementary Fig. 5D–F ), as well as levels of p53 mRNA ( Supplementary Fig. 5C ), were not significantly changed in the morphants studied. Cell clustering and multi-layering were dramatically impaired in the absence of fn1b , with few or no cells in the cardiac jelly in the majority of cases ( Fig. 7d,e ) indicating the importance of fibronectin deposition in the early stages of valve development. At 96 hpf, large groups of EdCs and reversing blood flow were visible in the AVC of fn1b MO embryos in contrast to the efficient valve leaflets present in controls ( Fig. 7f ). To confirm these observations, we analysed the valve shape of fn1b sa553−/− embryos at 96 hpf. Similar to fn1b knock down, we found that all the fn1b mutants had abnormal valves (9/9). The majority of these embryos displayed large blocks of cells occluding the AVC or thick leaflets as sometimes also described in the klf2a mutants ( Fig. 7g ). These data suggest klf2a and fn1b expression are necessary for the movement of EdCs into the cardiac jelly and their correct organization within. Thus mechanically-induced klf2a expression coordinates the morphogenetic events necessary for valve formation via the regulation of fibronectin1b expression and localized fibronectin synthesis within the AVC. 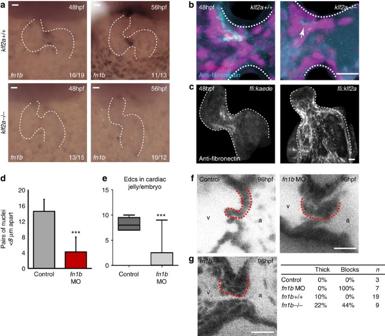Figure 7: Klf2a expression regulates fibronectin synthesis in the AVC to drive valve formation. (a)in situhybridization analysis shows thefn1bmRNA expression in the AVC ofklf2a+/+embryos, at 48 and 56 hpf, is lost in the majority ofklf2a−/−embryos. (b) Immunofluorescence analysis shows reduced fibronectin-positive staining (cyan) in the AVC ofklf2a−/−mutants (n=12klf2+/+,n=18klf2a−/−). Az-projection of the whole AVC is shown. (c) Forced expression of Klf2a in EdCs using theTg(fli:gal4FFubs; UAS:klf2a)line results in fibronectin-positive staining in the atrium and ventricle (n=12/16) compared with the AVC-specific staining pattern in controls (n=12/14) in at least three independent experiments. Az-projection of the whole heart is shown. (d) Analysis offn1bmorphants showed defective cell clustering in the superior AVC at 48 hpf (controln=6,fn1bMOn=5) and (e) reduced numbers of nuclei in the cardiac jelly at 72 hpf (controln=5,fn1bMOn=9). (f) Live imaging of valves at 96 hpf showed leaflets fail to form infn1bmorphants (controlsn=3,fn1bMOn=7). Single frames from the live imaging are shown and red dotted lines outline the superior valve leaflet in each case. The ventricle (v) and atrium (a) are labelled for orientation. (g) Single frames from the live imaging offn1b−/−mutant hearts, quantification of the percentage of thick/blocked valves observed infn1bMO,fn1b−/−mutant hearts and their respective controls. Student’st-test ***P<0.005, **P<0.01, *P<0.05. Scale bars, 10 μm. Figure 7: Klf2a expression regulates fibronectin synthesis in the AVC to drive valve formation. ( a ) in situ hybridization analysis shows the fn1b mRNA expression in the AVC of klf2a +/+ embryos, at 48 and 56 hpf, is lost in the majority of klf2a −/− embryos. ( b ) Immunofluorescence analysis shows reduced fibronectin-positive staining (cyan) in the AVC of klf2a −/− mutants ( n =12 klf2 +/+ , n =18 klf2a −/− ). A z -projection of the whole AVC is shown. ( c ) Forced expression of Klf2a in EdCs using the Tg(fli:gal4FF ubs ; UAS:klf2a) line results in fibronectin-positive staining in the atrium and ventricle ( n =12/16) compared with the AVC-specific staining pattern in controls ( n =12/14) in at least three independent experiments. A z -projection of the whole heart is shown. ( d ) Analysis of fn1b morphants showed defective cell clustering in the superior AVC at 48 hpf (control n =6, fn1b MO n =5) and ( e ) reduced numbers of nuclei in the cardiac jelly at 72 hpf (control n =5, fn1b MO n =9). ( f ) Live imaging of valves at 96 hpf showed leaflets fail to form in fn1b morphants (controls n =3, fn1b MO n =7). Single frames from the live imaging are shown and red dotted lines outline the superior valve leaflet in each case. The ventricle (v) and atrium (a) are labelled for orientation. ( g ) Single frames from the live imaging of fn1b −/− mutant hearts, quantification of the percentage of thick/blocked valves observed in fn1b MO, fn1b −/− mutant hearts and their respective controls. Student’s t -test *** P <0.005, ** P <0.01, * P <0.05. Scale bars, 10 μm. Full size image Using in vivo imaging technologies and cellular scale 3D analysis, we have identified three successive steps highlighting the cellular processes associated with heart valve morphogenesis: (1) the first signs of valve formation correspond to a regional increase in cell density in the superior AVC and localized fibrillogenesis; (2) the first sign of cellular invasion towards the cardiac jelly is highlighted by cell protrusions specifically in this area of cell clustering; and (3) a highly stereotyped multi-layering process within the cardiac jelly leading to the formation of a functional leaflet. These observations enable us to confirm the previously reported role of mechanical forces in valve morphogenesis [10] , [25] and suggest a refined model in which the origins of the valve progenitors, the behaviour of particular groups of cells and the impact of the mechanotransduction cascade are identified. Clustering of EdCs in a region of the AVC close to the ventricular inner curvature and localized fibronectin synthesis in the same area at 48 hpf is followed by the appearance of cells protruding into the cardiac jelly by 56 hpf. In the absence of klf2a , an important component of the mechanotransduction pathway downstream of blood flow [24] , cell clustering and fibrillogenesis are both impaired. Ultimately, the coordinated morphogenetic movements subsequently observed in control embryos are perturbed in klf2a mutants highlighting the importance of an intact mechanotransduction pathway in orchestrating the cellular events involved in valve formation. Interestingly, we observed a striking change in cell properties following migration into the cardiac jelly, with cells demonstrating a mesenchymal morphology, downregulating junctional Cdh5 and some of them proliferating. While we cannot rule out a contribution of cell proliferation in other parts of the heart driving cells towards the AVC, within the AVC itself we only observed cell proliferation within the cardiac jelly and not within the cell layer that is exposed to the blood flow. We demonstrated that flow forces primarily influence cell behaviour and ultimately valve shape, but not cell number, via the asymmetric activation of klf2a expression in the ventricular region of the AVC. Interestingly, klf2a −/− mutants presented an array of valvular phenotypes similar to those observed under a range of altered flow regimes, implicating Klf2a as an integrator of the flow response, which, when absent, impacts valvulogenesis from the earliest stages. It will be interesting to see if fibronectin also relays Klf2a function in other contexts, such as haematopoietic stem cells (HSC) formation [32] , development of the branchial arches [33] and endocardial chamber ballooning [6] . During valve formation the cells lining a unicellular tube are required to undergo extensive rearrangements in order to form a protrusive 3D structure capable of occluding undesired reversing flow. In the lymphatic system, the initial phases of valve formation have been elegantly described proceeding via the clustering of lymphatic valve progenitors on one side of the collecting vessel, adoption of a cuboidal morphology and the generation of a ring-like constriction within the vessel wall [11] . Valve-forming cells then protrude into the lumen of the lymphatic vessels, which, accompanied by ECM deposition, results in the formation of a valve leaflet [11] , [19] . In an initially similar manner, we see EdCs clustering on the ventricular side of the superior AVC, but rather than protruding towards the lumen, clustered EdCs then send basal protrusions into the cardiac jelly that they subsequently invade. These cells then proliferate and form a group of cells nestled close to the ventricular inner curvature, before a clear leaflet structure is formed. This significant difference in acquisition of cells into the leaflet in the lymphatic and cardiac systems is likely to be, at least in part, attributable to the different mechanical environments experienced by their progenitors. During cardiac valve formation in the mouse, EdCs within the AVC undergo an endothelial-to-mesenchymal transition (EMT) and migrate into the cardiac jelly [34] , where they proliferate and valve leaflets subsequently elongate. This is in striking contrast to lymphatic valve formation, which proceeds in the absence of an EMT. Interestingly, by embryonic day 10.5 (E10.5) the loss of klf2 results in AVC cell disorganization and hypocellular cushions, attributed to a defect in the EMT process [35] . We also observe AVC cell disorganization and, in some instances, hypocellular cushions in the absence of klf2a . Considering this together with the downregulation of Cdh5 by EdCs inside the cardiac jelly, cell morphology changes and increased proliferation, we hypothesize that the cellular protrusions observed from the clustered cells from 48 hpf and the subsequent movement of cells into the cardiac is reminiscent of the valve-forming process described in the mouse [35] . Importantly, the presence of an EMT during zebrafish valvulogenesis, although extensively discussed [18] , [26] , [28] , [36] , remains to be confirmed and will be an important focus of future studies. Valve morphogenesis occurs in one of the most hostile mechanical environments in the body: EdCs experience both high flow forces and strong mechanical deformation due to the contraction of the heart and its associated blood flow [1] . Indeed, at embryonic stages, viscosity dominates and the main mechanical forces generated at the heart wall are the tissue strain generated by pressure variations occurring during heart contraction and wall shear stress generated by the flowing blood [1] . These physical features are crucial to understanding how EdCs behave during valve development. Cell clustering close to the ventricular inner curvature in the AVC suggests localized differences in cell tension, which in turn may be responsible for the localized fibrillogenesis observed before multi-layering. The specific enrichment of klf2a expression in the AVC at 48 hpf in response to flow and its regulation of fibronectin1b expression provides a mechanism to modulate valve morphogenesis in response to its mechanical environment [25] . For now, we can only speculate on the role of fibronectin in the process of valve formation. One possibility is that fibronectin is necessary for EdCs to acquire a valvular cell fate as it is now becoming clear that forces, ECM and stem cells fate are tightly interdependent [37] . The discovery that the mechanical environment and stretch-sensitive channels are essential determinants of lineage choices in embryonic stem cells further supports this hypothesis [38] , [39] , [40] . Fibronectin could also be involved in promoting the generation of the filopodia observed at the onset of AVC-specific fibronectin accumulation and before the multi-layering process. Indeed, fibronectin-rich nanoenvironments have been demonstrated to be sufficient for orienting cell migration and proliferation [41] . In addition, fibronectin may alter the mechanical properties of the EdCs environment as well as several cellular properties, including the mechanosensitivity of the cells themselves. Fibronectin has been implicated in the endothelial mechanotranduction pathway mediated by trpv4 (ref. 42 ), a gene that is also involved in AVV formation [24] . Alternatively, fibrillogenesis could participate in cell-shape changes associated with morphogenesis [43] , a feature that has also been attributed to klf2a expression [6] . In conclusion, we propose a model for AVV formation in which EdCs arising from the atrium and ventricle make specific contributions to the emerging valve leaflets through coordinated cell-movement events. Enriched mechanosensitive klf2a expression on the ventricular side of the AVC subsequently enriches the expression of its downstream target gene fibronectin1b to the same cells, establishing an asymmetry within the AVC. Ventricular EdCs extend protrusions towards the fibronectin-rich area and move into the cardiac jelly in a coordinated manner while accompanying morphogenetic changes result in atrial EdCs lining the lumen of the AVC. Subsequent Cdh5-downregulation, increased proliferation and morphological changes within the AVC liken aspects of AVV formation in the zebrafish to that of the mouse and higher vertebrates. Finally, this study elucidates the impact of mechanical forces on the localized behaviours of valve progenitors during valve morphogenesis. As the origins of most valvulopathies are still unknown [12] , our findings highlight the importance of investigating the potential embryonic and mechanical origins of valve defects. The recent demonstration that mitral valve disease can have embryonic origins supports this view [44] , [45] , [46] . Furthermore our work highlights the role of the coordination between morphogenesis and mechanical forces via ECM synthesis during cardiovascular morphogenesis. These findings may also prove meaningful in other biological contexts where mechanical forces and ECM are involved, such as during stem cell niche formation in developing HSCs [47] , [48] , [49] , skin stem cells [50] and adult intestinal stem cells [51] . Zebrafish husbandry, embryo treatments and morpholinos Animal experiments were approved by the Animal Experimentation Committee of the Institutional Review Board of the IGBMC. Zebrafish lines used in this study were Tg(fli1a:gal4FF ubs ; UAS:kaede) [52] , Tg(fli1a:nEGFP) y7 (ref. 53 ) , Tg(kdrl:EGFP) [54] , Tg(fli:nls-mcherry) [24] , Tg(myl7:EGFP) [55] , Tg(fli:gal4FF ubs ; UAS:klf2a) (ref. 6 ), Tg(klf2a:H2BEGFP) [24] and wild-type AB. Zebrafish with a mutant allele of klf2a (Tg(klf2a ig4 )) were generated and used in this study. Zebrafish with a mutant allele of fn1b (Tg(fn1b Sa553 ) were obtained from the Zebrafish International Resource Center (ZIRC). Tg(fn1b Sa553 ) mutants contain a C>T point mutation in exon 1 of the fn1b gene leading to a premature stop codon in the predicted translation product. Genotyping was performed by sequencing the PCR product generated with the following primers: forward 5′- AGGGTGAGAGAACCTCATAAAGC -3′, reverse 5′- CTCACTTAAACCGCGAACTGTCC -3′, and sequenced with 5′- TCAGTAAAGAGACTCCTGCTGC -3′. Genotyping was performed on genomic DNA after live imaging. Morpholinos were injected into the yolk at the one-cell stage. All animals were incubated at 28.5 °C for 5 h before treatment with 1-phenyl-2-thiourea (PTU) (Sigma Aldrich) to prevent pigment formation. Morpholinos specific for tnnt2a (ref. 30 ) (5′- CATGTTTGCTCTGATCTGACACGCA -3′) and fn1b (5′- AAGTAATAATGTCACCTTGCTCCTC -3′) were obtained from GeneTools. Morpholinos for klf2a , gata1, gata2 and myh6 were described previously [25] , [56] . Anti-sense MO concentrations ranged from 0.06 to 0.3 mM. Generation of klf2a −/− mutants We injected a TALEN pair designed to target exon 1 of the klf2a gene into single cell wild-type (AB) embryos. We identified the alleles generated and confirmed that potential targeting events could be transmitted through the germline by out-crossing the F0 fish with AB animals and sequencing genomic DNA from pools of 6 F1 embryos. We focused on an INDEL mutation (deletion of 5′- CAGAAGGAA -3′ followed by insertion of 5′- GATGCTGGGAGAG -3′) leading to a premature stop codon in the klf2a transcript and raised these F1 animals to adulthood. Studies were performed on F2 fish, and later generations, following out-crossing to transgenic lines of interest. Klf2a −/− fish were viable and also kept as homozygous adults. A PCR-based genotyping strategy was established using the following primers to identify the wild-type and mutant alleles (Wild-type: forward 5′- TCGGCGCAGAAGGAAA -3′, reverse 5′- TGTTGAGGTTGTCCATGTTA -3′; mutant: forward 5′- AAGGTCTTCCACCACTCATA -3′, reverse 5′- CCAGCATTTCTCTCCCAGC -3′). Genotyping was performed on genomic DNA from whole embryos after live imaging, or from dissected tails before immunofluorescence analysis, as necessary. mRNA sequencing of dissected heart samples Hearts were dissected from Tg(myl7:EGFP) embryos at the desired stage and pooled (30 hearts/sample). RNA was extracted using a Nucleospin RNA XS kit (Macherey-Nagel) according to the manufacturer’s instructions. After isolation of total cellular RNA, a library of template molecules suitable for high throughput DNA sequencing was created following the Illumina ‘mRNA sequencing sample preparation guide’ (part #1004898 Rev.D) with some modifications. Briefly, mRNA was purified from 20 ng total RNA using oligo-dT magnetic beads and fragmented using divalent cations at 94 °C for 5 min. The cleaved mRNA fragments were reverse transcribed to cDNA using random primers, then the second strand of the cDNA was synthesized using DNA Polymerase I and RNase H. The next steps of RNA-Seq Library preparation were performed in a fully automated system using SPRIworks Fragment Library System I kit (ref A84801, Beckman Coulter, Inc) with the SPRI-TE instrument (Beckman Coulter, Inc). Briefly, in this system, double-stranded cDNA fragments were blunted, phosphorylated and ligated to indexed adapter dimers, and fragments in the range of ∼ 200–400 bp were size selected. The automated steps were followed by PCR amplification (30 s at 98 °C; (10 s at 98 °C, 30 s at 60 °C and 30 s at 72 °C) × 13 cycles; 5 min at 72 °C), then surplus PCR primers were removed by purification using AMPure XP beads (Agencourt Biosciences Corporation). DNA libraries were checked for quality and quantified using a 2100 Bioanalyzer (Agilent). The libraries were loaded in the flow cell at 6 pM concentration and clusters generated and sequenced in the Illumina Genome Analyzer IIX as single-end 54 base reads. The data discussed in this publication have been deposited in NCBI's Gene Expression Omnibus [57] and are accessible through GEO Series accession number GSE79585 ( https://www.ncbi.nlm.nih.gov/geo/query/acc.cgi?acc = GSE79585). Bioinformatics and gene ontology analysis Read quality was assessed with FastQC (S. Andrews, http://www.bioinformatics.babraham.ac.uk/projects/fastqc/ ). Then reads were mapped onto the Zv9 assembly of the zebrafish genome using Tophat v1.4.1 (ref. 58 ) and the bowtie v0.12.7 aligner. Only uniquely aligned reads were retained for further analyses. Gene expression was quantified using HTSeq v0.5.3p5 (ref. 59 ) and gene annotations from Ensembl release 69. Read counts were normalized across libraries with the method proposed by Anders et al . [60] . To identify significantly differentially expressed genes, we performed a test for differential expression within the experiment (that is, adjusting for baseline differences between the experiments) using the method proposed by Robinson and Smyth [61] and implemented in the Bioconductor edgeR v3.0.8 package [62] . Adjustment for multiple testing was performed with the Benjamini and Hochberg [63] method. Functional analyses of genes with an adjusted P value smaller than 0.05 were performed using DAVID software [64] . Graphics were obtained with the R program (R Core Team, URL http://www.R-project.org/ ). qPCR Products were amplified in a real-time PCR reaction with Light Cycler 480 Real-Time PCR System (Roche) using a UPL Probes Master mix (Roche) according to the manufacturer’s instructions. Sequence of primer pairs were as follows: has2 forward 5′- AGCATCCCTGTTCAACTAACG -3′, reverse 5′- GCTGACCGCTTTATCACATCT -3′ ; klf2a forward 5′- CCGTCTATTTCCACATTTTCG -3′, reverse 5′- TCCAGTTCATCCTTCCACCT -3′; fn1b forward 5′- TGGAAATGTGATGCCATTGA -3′, reverse 5′- GGCCAATCTGGTAGAACACC -3′; p53 forward 5′- GAGGTCGGCAAAATCAATTC -3′, reverse 5′- TGGGGGCTGAATAATCAAAT -3′. In vivo imaging Zebrafish embryos were staged, anaesthetised with 0.02% tricaine solution and 50 mM BDM, to stop the heart when necessary, and mounted in 0.7% low melting-point agarose (Sigma Aldrich). Confocal imaging was performed on a Leica SP8 confocal microscope. Fast confocal and four-dimensional imaging (to image valve leaflets at 96 hpf and the AVC at 72 hpf) was performed using the resonant scanner mode of the same microscope. Images were acquired with a low-magnification water immersion objective (Leica HCX IRAPO L, 25X, N.A. 0.95). For four-dimensional imaging, time series were acquired at a random time in the cardiac cycle at 35fps for 3 s. The optical plane was moved 2 μm between the z -sections until the whole AVC was acquired. Time series of two-dimensional sections were temporally synchronized using Matlab [27] . Blood flow imaging for flow velocity analysis was performed on a Leica DMIRBE inverted microscope using a Photron SA3 high speed CMOS camera (Photron, San Diego, CA) and water immersion objective (Leica × 20, NA 0.7). Image sequences were acquired at a frame rate of 2,000 frames per second. Photoconversion Photoconversion was performed using the FRAP module on a SP8 confocal microscope and a Leica HCX IRAPO L, × 25, NA0.95 water immersion objective. Tg(fli1a:Gal4FF; UAS:Kaede) embryos were mounted in 0.7% low melting-point agarose supplemented with 50 mM BDM to inhibit heart contraction for the duration of the procedure. A region of interest corresponding to the ventricle, atrium or superior AVC was selected and exposed to 405 nm light (25% laser power). One pre-bleach frame was acquired, followed by 3–5 bleach pulses (3–5 ms each) without acquisition to achieve conversion of the kaede protein to its red form. A z -stack of the photoconverted heart was then acquired in the standard confocal mode to record the starting point of each experiment. Embryos were then carefully dissected from the agarose, placed in fish water for 5–10 min until heart contraction resumed and then put at 28.5 °C to develop individually under standard conditions until a time point of interest. The movement of cells within each heart was analysed using Imaris software (Bitplane). Valve imaging Embryos were incubated with 4 μM BODIPY-ceramide (Molecular Probes) overnight and then processed as in refs 24 , 25 to visualize the valve shape. Flow analysis Red blood cells were manually tracked through the AVC and their velocity calculated from image sequences acquired at 2,000 frames per second as described previously [24] . Immunofluorescence Embryos were fixed at the desired stage in 2% paraformaldehyde overnight at 4 °C. BrdU-incorporation studies were performed by incubating embryos in 5 mg ml −1 BrdU for the desired length of time (Dietrich et al . [6] ) before fixation. After washing, embryos were permeabilized in 1 × PBS-0.1% Tween-20 containing 0.5% Triton-X 100 for 30 min at room temperature. The pericardial cavity was then carefully pierced with the tip of a forcep to facilitate antibody penetration before blocking in permeabilization buffer supplemented with 5% BSA (anti-fibronectin), 1% BSA and 10% NGS (anti-VECadherin and anti-Alcama) or 1% BSA, 2% NGS and 1% DMSO (anti-BrdU) for 2 h at room temperature. Primary antibodies were added in the relevant blocking solution and incubated between 16 and 48 h at 4 °C. Secondary antibodies were added in blocking solution after thorough washing and incubated overnight at 4 °C. Embryos were thoroughly washed and mounted for imaging on a Leica SP8 confocal. Antibodies were as follows: rabbit anti-fibronectin (F3648, Sigma) 1:100, rabbit anti-VECadherin [65] 1:1,000 (kind gift of the Affolter lab), mouse anti-BrdU (11170376001, Roche Diagnostics) 1:100, mouse anti-Alcama (zn-8, DSHB) 1:500 and goat anti-rabbit and goat anti-mouse Alexa-488 and -594 secondary antibodies (A11034 and A11032, respectively, Life Technologies) were used at 1:500. To directly test the effects of flow on fibronectin synthesis, embryos were incubated in 0.1% tricaine (Ethyl 3-aminobenzoate methanesulfonic acid; Sigma) at pH7 for up to 12 h. They were then rinsed briefly in egg water before being fixed and processed as described above. Cell proliferation assay Dechorionated embryos were incubated in fish water containing 5 mg ml −1 BrdU between 36 and 48 hpf, 56 and 72 hpf, and 72 and 80 hpf. Incorporation was stopped by washing in fresh fish water and fixation in 4% PFA. Embryos were permeabilized with Proteinase K and DNA denatured with 2 N HCl (method modified from Dietrich et al . [6] ). BrdU immunolabelling was then performed as described above. Image analysis Cell number quantifications and klf2a : EGFP signal intensity measurements were made using the Spots tool on Imaris (Bitplane). A single spot was placed at the centre of each nucleus in the AVC, or cardiac jelly, as appropriate. For intensity analysis, the klf2a:H2BEGFP reporter line was crossed with the fli:nlsmCherry line and the mCherry fluorescence signal was used for normalization [24] . The maximum intensity of each channel was quantified and a ratio generated. These ratios were then averaged across the AVC of individual embryos. Nucleus to nucleus distance analysis was performed using Imaris software and the Measurement Points tool. Nuclei within the AVC were connected to all of their nearest neighbours and the average distances for defined regions were calculated. The extent of cell clustering, in klf2a mutants and fn1b morphants, was quantified by defining clustered cells as those cells closer than 8 μm to their neighbour (according to our analysis of nucleus-to-nucleus distances in controls; Fig. 2e ). The extent of fibronectin staining in the AVC was calculated using the Imaris Surfaces tool to define a volume of fibronectin staining and a volume of the whole AVC. The % of fibronectin coverage was then calculated ([Volume fibronectin staining/Volume AVC]*100). Hearts were segmented using the surfaces tool and the segmented heart presented, for clarity. In situ hybridization In situ hybridization was performed as in ref. 66 . Anti-sense probes for fn1b were generated from a plasmid containing fn1b cDNA (obtained from SourceBioscience) amplified using the following primers forward: 5′- ATGACCCGTGAGTCAGTAA -3′ and reverse (containing T3 sequence): 5′- ATTAACCCTCACTAAAGGGACTTGGTGCCCTGAGTTCTGAT -3′ and subsequently transcribed using the T3 polymerase. Accession codes: The gene expression data have been deposited in the NCBI Gene Expression Omnibus (GEO) database under accession code GSE79585 . How to cite this article: Steed, E. et al . klf2a couples mechanotransduction and zebrafish valve morphogenesis through Fibronectin synthesis. Nat. Commun. 7:11646 doi: 10.1038/ncomms11646 (2016).